Fluidic supramolecular nano- and microfibres as molecular rails for   regulated movement of nanosubstances Nano- and micro-sized fibrous architectures are ubiquitous in nature; in particular,    microtubules have an essential role within live cells, as tracks for transporting objects to    a desired place, driven by molecular motors such as dynein and kinesin. Such functions of    bionanofibres motivated us to construct an artificial supramolecular rail using the fluidic    property of self-assembled glycolipid nanofibres. Artificial supramolecular nanofibres    constructed through molecular self-assembly of small molecules have recently attracted    considerable attention for their unique properties, such as reversible formation/destruction    under mild conditions and various stimuli responsiveness. In this paper, we show that a    supramolecular nanofibre has sufficient fluidity, on the basis of its non-crystalline    nature, to function as a molecular track for the directional movement of attached molecules,    proteins and nanobeads along the fibre. Substances having well-defined fibrous nanostructures are anticipated as key materials for   developing sophisticated electrical, chemical or biological devices in nanotechnology [1] , [2] , [3] , [4] , [5] , [6] , [7] , [8] . Carbon nanotubes [9] are a representative   fibrous nanomaterial, not only in nanoelectronic devices such as an electric wire, a   capacitor, a transistor or an emitter of field emission display but also in nanomechanics as a   probe for a scanning tunneling microscope or atomic force microscope [10] . As   alternatives to the carbon nanotube, self-assembled fibrous architectures have recently been   developed by bottom-up technology. For instance, a nanotube comprising an amphiphilic    hexabenzocoronene derivative   was reported to show high electric conductivity through a crystalline π-stacked graphitic    layer [7] , [8] . Supramolecular nanofibres were also elegantly used as templates   for synthesis of inorganic nanomaterials [11] , [12] . Apart from the use of   crystalline nanofibres, dynamic and flexible properties such as fluidity should be one of the   unique and essential features of supramolecular fibres, although these have been   insufficiently explored. In nature, indeed, flexible self-assembled bionanofibrils have   important roles for in-cell molecular transportation systems, cell migration and other dynamic    phenomena [13] . For example, natural motor proteins such as myosin, kinesin or   dynein walk along bionanofibrils (actin filaments or microtubules) unidirectionally, under   conditions in which Brownian motion and viscous forces are dominant, using the chemical energy   derived from ATP hydrolysis   (50–60 kJ mol −1 or ∼ 22 k B T, where k B is the Boltzmann constant) [14] , [15] , [16] . Recent   studies have emphasized the importance of Brownian motion (diffusive component, such as   diffusional search process of the free motor domain head), as well as rigid conformational   changes (mechanical component) of motor proteins coupled with ATP hydrolysis for such efficient   one-directional transport [17] , [18] , [19] . Very recently, an increasing number of   microtubule-binding proteins have been found to exhibit diffusional motility along the   microtubule lattice (one-dimensional random walk) [20] , [21] , which did not require    ATP and is thus regarded as   an economical mode of transport. Similar one-dimensional diffusive motion without    ATP hydrolysis was observed   for a DNA-binding protein moving along the DNA fibre [22] , [23] . However, the   proportion and importance of the diffusive component contribution into the one-dimensional   transport is still controversial. The construction of simple artificial supramolecular   rail-cargo systems on a micrometre scale is expected to provide appropriate models for deep   understanding of the role of the diffusive component in one-directional motion and thus give a   clue for building a well-developed mass transport network. However, limited knowledge is   currently available for artificial supramolecular machinery systems that can work on scales   (submicro to micrometre), which are comparable with biological systems [24] , [25] , [26] , [27] , [28] . In contrast, many elegant synthetic molecular machines have   emerged on the nanometre scale, especially in the field of supramolecular chemistry [29] , [30] , [31] , [32] , [33] , [34] , [35] , [36] , [37] , [38] . Molecular design of supramolecular fibres as molecular rails We have recently been interested in the hydrogel formation of a self-assembled     supramolecular nanofibre in an aqueous solution composed of glycosylated L -glutamate esters bearing two     tails, such as n -hexyl ( 1 ) or methyl-cyclohexyl ( 2 ) groups [39] , [40] , [41] , [42] ( Fig. 1a ). Here, we showed that the gel     state is completely distinctive from the crystalline state in terms of fibre fluidity. Using the fluidity, we showed that mixed gelator-like molecules ( 3 , 4 and 5 , see Supplementary Method ) were     transported along nanofibre 1 . In particular, the biotin-tethered gelator mimic 5 was spontaneously mixed to form functionalized nanofibres 1 / 5 ( Supplementary Fig. S1 ) that can work as a     molecular rail to guide the movements of attached avidin protein and avidin-coated     nanobeads in the range of nanometres to tens of micrometres ( Fig. 1b,c ). 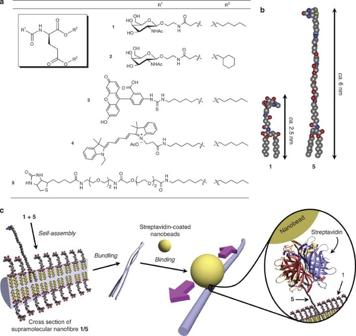Figure 1: Supramolecular nanofibre as a molecular rail for nanobeads. (a) Chemical structures of lipid-like molecules1,2,       FITC-lipid (3),      Cy5-lipid (4) and Biotin-lipid (5). (b) Molecular models of lipids1and5. (c) Schematic showing self-assembly of lipids1and5into a supramolecular nanofibre and binding of nanobeads to the fibre      through a biotin–avidin      interaction, which results in regulated one-dimensional motion. Figure 1: Supramolecular nanofibre as a molecular rail for nanobeads. ( a ) Chemical structures of lipid-like molecules 1 , 2 ,       FITC-lipid ( 3 ),      Cy5-lipid ( 4 ) and Biotin-lipid ( 5 ). ( b ) Molecular models of lipids 1 and 5 . ( c ) Schematic showing self-assembly of lipids 1 and 5 into a supramolecular nanofibre and binding of nanobeads to the fibre      through a biotin–avidin      interaction, which results in regulated one-dimensional motion. Full size image Morphology and fluidic property of supramolecular nanofibres Transmission and scanning electron microscopic (TEM and SEM) observations of nanofibre 1 revealed high-aspect-ratio fibres with a 10–100 nm range in diameter ( Supplementary Fig. S2a,b ). A confocal     laser-scanning microscopic (CLSM) image also showed fibrous networks stained by      1-anilinonaphthalene-8-sulphonic      acid (ANS), an environmentally sensitive fluorescent probe, suggesting that     incipient, thin nanofibres bundled together to form thick microfibres and that the present     nano/microfibre contains a well-developed continuous hydrophobic domain ( Supplementary Fig. S2c ). Interestingly, various     morphologies of nanofibre 1 emerged, such as tangled ropes, coiled and wavy fibres      ( Fig. 2a–c ). Moreover, nanofibre 1 can be aligned in a     microfluidic channel created by poly(dimethylsiloxane) (PDMS). Figure      2d,e shows the morphological change of nanofibre 1 before and after the     application of electric voltage (50 V cm −1 ) in a microchannel of PDMS (150     μm in width×50 μm in depth), respectively. This result shows that nanofibre 1 has     sufficient elastic toughness and flexibility for aligning in microchannels under the     application of electric voltage or laminar flow ( vide infra ). 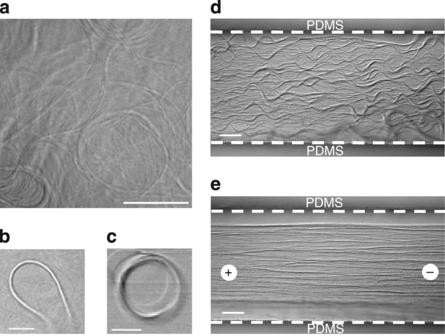Figure 2: Morphological variety of supramolecular nanofibre1observed by CLSM. (a–c) Various lariat- and coil-shaped nanofibres1(1=0.25      wt% (3.8 mM)). (d,e) Nanofibre1in a microfluidic PDMS      (poly(dimethylsiloxane)) device as introduced (d) and linearly aligned by      electric field (e) (1=0.25 wt%, 100 mM      Tris(tris(hydroxymethyl)aminomethane)–HCl buffer (pH 7.4)). The fields of vision for      imagesdandewere the same and imagedwas obtained by applying      voltage at 50 V cm−1. All images were acquired in differential      interference contrast (DIC) mode. The scale bars ina–eare 10, 5, 10, 30      and 30 μm. Figure 2: Morphological variety of supramolecular nanofibre 1 observed by CLSM. ( a – c ) Various lariat- and coil-shaped nanofibres 1 ( 1 =0.25      wt% (3.8 mM)). ( d , e ) Nanofibre 1 in a microfluidic PDMS      (poly(dimethylsiloxane)) device as introduced ( d ) and linearly aligned by      electric field ( e ) ( 1 =0.25 wt%, 100 mM      Tris(tris(hydroxymethyl)aminomethane)–HCl buffer (pH 7.4)). The fields of vision for      images d and e were the same and image d was obtained by applying      voltage at 50 V cm −1 . All images were acquired in differential      interference contrast (DIC) mode. The scale bars in a – e are 10, 5, 10, 30      and 30 μm. Full size image The fluorescence recovery after photobleaching (FRAP) experiments [43] gave     an insight into the dynamic property of nanofibre 1 . Fluorescein isothiocyanate      (FITC)-lipid 3 was used as a probe molecule, because FITC derivatives can be easily photobleached by an intense Ar laser     light (488 nm) equipped with CLSM. After the irradiation of the intense laser light to a     lariat-shaped nanofibre 1 , the fluorescence image at the same field of vision was     continuously monitored in real time. 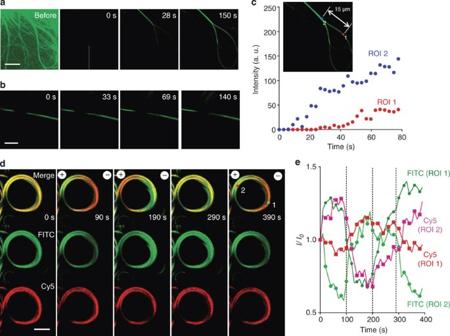Figure 3: Fluidic property of supramolecular nanofibre1evaluated by FRAP experiment     and electrically regulated transport of ionic fluorescent lipids along the fibre. (a,b) Time-lapse CLSM images for nanofibres1/3(a)      and2/3(b) after photobleaching. (c) Plots of fluorescence      intensity depending on time for nanofibres1/3at marked regions ROI      (region of interest)1,2in the inset ofc. (1=0.25 wt%,2=0.25 wt%, FITC-lipid3=3.0 μM in 50 mM HEPES (4-(2-hydroxyethyl)-1-piperazineethanesulfonic       acid) buffer (pH 7.2)). (d) CLSM images of coil-shaped      nanofibres1/3+4during the sequentially applied electric voltage.       (e) Plots of fluorescence intensity depending on time at marked ROI 1, 2 shown      in the image ofd(merge,t=390 s) (1=0.25 wt%, agarose=2.0 wt%,       FITC-lipid3=3.0 μM, Cy5-lipid4=6.0 μM in 50 mM HEPES buffer (pH 7.2); applied      voltage, 15 V cm−1). Dotted lines denote times when the voltage direction      was switched or voltage was cutoff. The scale bars ina,banddare 10, 50 and 10 μm, respectively. As shown in Figure 3a, the     bleached dark area became bright so that the FITC fluorescence recovered along the     original fibre shape within 50 s because of the rapid supply of non-bleached 3 to     the bleached region from the non-bleached edge, which clearly indicates that nanofibre 1 possesses fluidity and is structurally continuous at least up to several tens     of micrometres. In sharp contrast, such a fluorescence recovery has never been observed in     the case of self-assembled crystalline fibre 2 , an analogue of 1 bearing     more hydrophobic cyclohexyl groups instead of n -hexyl groups, indicating that fibre     fluidity was completely suppressed in the crystalline state ( Fig. 3b ). Figure 3c shows the typical time profile of the     fluorescence recovery process for two different positions on the same fibre (marked as     region of interest (ROI) 1 and ROI 2 in Fig. 3c ), with a separation     of 15 μm. The fluorescence recovery at ROI 1 was delayed by 18 s relative to that at ROI     2, the value of which gave us the lateral diffusion speed ( v ) of lipids on the     supramolecular fibre. The averaged value of lateral diffusion speed ( v ) was     estimated to be 0.7±0.2 μm s −1 from seven independent experimental     measurements. It was previously reported that the diffusion coefficient ( D ) of lipid molecules in biomembranes in aqueous solution at 25 °C is ∼ 1.0 μm 2 s −1 (ref. 44 ), which gives a root mean     square (r.m.s.) distance (2 Dt ) 1/2 =2.0 μm during a delay of 1.0 s.     Thus, the fluidity of the supramolecular nanofibre 1 is slightly lower than that of     biomembranes. Figure 3: Fluidic property of supramolecular nanofibre 1 evaluated by FRAP experiment     and electrically regulated transport of ionic fluorescent lipids along the fibre. ( a , b ) Time-lapse CLSM images for nanofibres 1 / 3 ( a )      and 2 / 3 ( b ) after photobleaching. ( c ) Plots of fluorescence      intensity depending on time for nanofibres 1 / 3 at marked regions ROI      (region of interest) 1 , 2 in the inset of c . ( 1 =0.25 wt%, 2 =0.25 wt%, FITC-lipid 3 =3.0 μM in 50 mM HEPES (4-(2-hydroxyethyl)-1-piperazineethanesulfonic       acid) buffer (pH 7.2)). ( d ) CLSM images of coil-shaped      nanofibres 1 / 3 + 4 during the sequentially applied electric voltage. ( e ) Plots of fluorescence intensity depending on time at marked ROI 1, 2 shown      in the image of d (merge, t =390 s) ( 1 =0.25 wt%, agarose=2.0 wt%,       FITC-lipid 3 =3.0 μM, Cy5-lipid 4 =6.0 μM in 50 mM HEPES buffer (pH 7.2); applied      voltage, 15 V cm −1 ). Dotted lines denote times when the voltage direction      was switched or voltage was cutoff. The scale bars in a , b and d are 10, 50 and 10 μm, respectively. Full size image Regulated transport of ionic lipids along supramolecular nanofibres The fluidity of nanofibre 1 was further confirmed by an electrically controlled     localization change of the ionic probes on it. A cationic fluorescent probe, cyanine     5-lipid 4 , was embedded in nanofibre 1 , together with anionic      FITC-lipid 3 . Figure 3d shows typical CLSM images of a coiled fibre during     sequential application of electric voltage, in which emissions from 3 and 4 are coloured green and red, respectively. Without voltage application, the colour of the     whole fibre is uniformly yellow, which is a perfectly merged colour of green and red,     indicating the homogeneous distribution of 3 and 4 within the coiled fibre. Under applied voltage, the green emission from 3 gradually moved and concentrated     at the cathode (left) side of the fibre, whereas the red emission from 4 concurrently moved to the anode (right) side. After 90 s, these two emission areas were     distinctively segregated within different fibre domains, indicating that cationic 4 and anionic 3 are heterogeneously localized at the anode and cathode sides of the     coiled fibre, respectively. The distribution of 3 and 4 on the fibre was     reversibly replaced by one another by switching the direction of the applied voltage (190     s, left: anode, right: cathode), and the biased distribution was readily relaxed by     cutting off the voltage (290 s). Figure 3e shows the profiles for     the fluorescence intensity change of 3 and 4 at the marked region of the     fibre. It is clear that the fluorescence intensity of 3 decreased and then     increased by switching the voltage direction, the behaviour of which was sharply in     contrast to that of 4 in each region. These results show that ionic molecules     embedded in the supramolecular fibre can be transported along the fibre by an external     voltage, depending on the charge of the molecules, because of fibre fluidity. Regulated motion of nanobeads on supramolecular rails To trace the motion of a single molecule along the fluidic supramolecular nanofibre     directly and individually by microscopy, we next used nanoparticles as probes. Nanoparticle tracking has been recently used to evaluate the motion speed of nanoparticles     attached to fluidic membranes [45] , [46] , [47] or biomolecular motor [48] , [49] until hydrodynamic friction against larger nanoparticles set the upper     limit for the motion speed. To attach nanoparticles to fibres, we modified the molecular     recognition property of supramolecular nanofibre 1 with biotin-lipid 5 ( Fig. 1c , Supplementary Fig. S1 ). First, CLSM observations revealed that nanofibres 1 / 5 can bind a     streptavidin (SA) protein labelled with fluorescence dyes ( Supplementary Fig. S3 ). In addition, the lateral diffusion of the SA     protein bound to nanofibres 1 / 5 was evidenced by FRAP experiments using      FITC-labelled SA ( Fig. 4a,b , Supplementary Fig. S4 ), which afforded an averaged diffusion coefficient ( D ) of 0.12±0.03      μm 2 s −1 at 25 °C. From the diffusion coefficient, the     r.m.s. distance (2 Dt ) 1/2 during a delay of 1.0 s was estimated to be     0.5 μm, which is comparable with the value of the lateral diffusion speed of lipids on     supramolecular fibre 1 . In addition, the FRAP recovery percentage reached ∼ 90% ( Fig. 4b ). These data indicate that the binding of SA to      biotin-lipid 5 in     supramolecular nanofibre 1 did not destroy the continuous structure of the fibres. In contrast, self-assembled fibres 2 / 5 were able to bind SA but did not show     lateral diffusion of the bound SA, which is consistent with the data of Fig. 3a,b (data not shown). We then traced the motion of three different sizes     of nanobeads coated with SA (50, 250 and 500 nm in diameter), which successfully attached     to nanofibres 1 / 5 through an avidin–biotin interaction ( Supplementary Figs. S5–7 ). Most interestingly,     by careful examination of the time-lapsed CLSM images and movies, one-dimensional motions     of the bound SA beads along the long axis of nanofibres 1 / 5 were captured at     a single molecular level ( Fig. 4c , also see Supplementary Movie 1 ). Such a one-dimensional     motion was not observed for control experiments using nanofibre 1 and SA beads     (that is, in the absence of 5 ), or nanofibres 1 / 5 and SA beads in the     presence of excess biotin     (that is, with the biotin-binding site of SA masked) ( Supplementary Figs. S5–7 ). 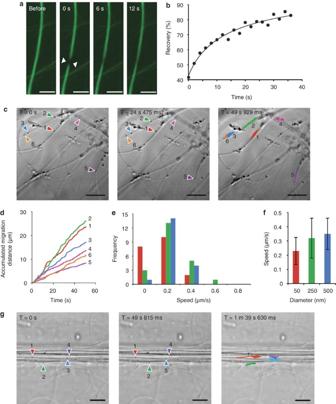Figure 4: Regulated motions of nanobeads on supramolecular nanofibres1/5. (a) Time-lapse CLSM images for nanofibres1/5binding       FITC-labelled SA after      photobleaching. (b) Fluorescence recovery curve with a one-dimensional diffusion      model fit (Supplementary Fig. S4)      (1=0.10 wt%, biotin-lipid5=24 μM (1.6 mol% against1),       FITC-labelled SA=18 μg       ml−1). (c) Time-lapse CLSM images (DIC mode) of nanofibres1/5attaching 250-nm SA beads. The trace merged in the right panel      denotes the directed motion of the SA beads along the long axis of the nanofibres (Supplementary Movie 1). (d) Time      courses of the accumulated migration distances of 250 nm SA beads at 25 °C corresponding      toc. (e) Histograms of average lateral diffusion speeds of 50 nm (red, 20      individual beads), 250 nm (green, 22 individual beads) and 500 nm (blue, 19 individual      beads) SA beads at 25 °C evaluated from the series of time-lapse CLSM images (Supplementary Fig. S8). (f) Averaged      lateral diffusion speeds depending on the diameter of SA beads. (g) CLSM images      (DIC mode) of nanofibres1/5attaching 250 nm SA beads in a microchannel      fabricated by PDMS (50 μm in height, 300 μm in width). The trace merged in the right      panel denotes the directed motion of 250 nm SA beads along the nanofibres (Supplementary Movie 2) (1=0.10 wt%,       biotin-lipid5=24 μM (1.6 mol% against1)). The scale bars ina,candgare 5 μm. Figure 4: Regulated motions of nanobeads on supramolecular nanofibres 1 / 5 . ( a ) Time-lapse CLSM images for nanofibres 1 / 5 binding       FITC-labelled SA after      photobleaching. ( b ) Fluorescence recovery curve with a one-dimensional diffusion      model fit ( Supplementary Fig. S4 )      ( 1 =0.10 wt%, biotin-lipid 5 =24 μM (1.6 mol% against 1 ),       FITC-labelled SA=18 μg       ml −1 ). ( c ) Time-lapse CLSM images (DIC mode) of nanofibres 1 / 5 attaching 250-nm SA beads. The trace merged in the right panel      denotes the directed motion of the SA beads along the long axis of the nanofibres ( Supplementary Movie 1 ). ( d ) Time      courses of the accumulated migration distances of 250 nm SA beads at 25 °C corresponding      to c . ( e ) Histograms of average lateral diffusion speeds of 50 nm (red, 20      individual beads), 250 nm (green, 22 individual beads) and 500 nm (blue, 19 individual      beads) SA beads at 25 °C evaluated from the series of time-lapse CLSM images ( Supplementary Fig. S8 ). ( f ) Averaged      lateral diffusion speeds depending on the diameter of SA beads. ( g ) CLSM images      (DIC mode) of nanofibres 1 / 5 attaching 250 nm SA beads in a microchannel      fabricated by PDMS (50 μm in height, 300 μm in width). The trace merged in the right      panel denotes the directed motion of 250 nm SA beads along the nanofibres ( Supplementary Movie 2 ) ( 1 =0.10 wt%,       biotin-lipid 5 =24 μM (1.6 mol% against 1 )). The scale bars in a , c and g are 5 μm. Full size image The averaged lateral diffusion speed ( v ) of the bound beads was estimated to be     0.23±0.095 μm s −1 for 50 nm, 0.32±0.14 μm s −1 for 250 nm and     0.35±0.11 μm s −1 for 500 nm beads from a plot of accumulated migration     distance against time ( Fig. 4d ), which approximately showed Gaussian     distributions ( Fig. 4e ). The obtained lateral diffusion speeds were     almost independent of bead size and were comparable with those of lipid molecules in the     nanofibres and the FITC-SA     protein bound to the nanofibres ( Fig. 4f ). These results strongly     support the view that the lateral diffusion of beads bound to nanofibre 1 is     predominantly regulated by the fluidity of the fibre. These values are almost one order of     magnitude lower than those for free spheres in water, calculated on the basis of the     Stokes–Einstein equation. Moreover, these values are comparable with those for 30 nm     nanogold-coated anti-flourescein (0.26 μm 2 s −1 ), which was     attached to fluorescein-conjugated phosphatidylethanolamine in a supported bilayer      membrane [45] , and vesicles (30–200 nm in diameter, typically 0.2      μm 2 s −1 ) attached to a DNA–lipid conjugate by DNA     hybridization in a supported bilayer membrane [46] . The latter particles     showed two-dimensional random motion on the substrates, which was independent of vesicle     size, because of the fluidity of the membrane. In addition, supported bilayer membrane     systems require fabricated template materials and tedious procedures under rigidly     controlled conditions to construct the one-dimensional systems [50] , [51] , [52] , [53] . By simply aligning nanofibres 1 / 5 parallel with the long axis of a     microchannel using laminar flow, the motion of the bound nanobeads became directional, in     unison along the long axis of the aligned nanofibres 1 / 5 ( Fig. 4g , see also Supplementary Movie      2 ). The lateral diffusion speed of the bound nanobeads was evaluated to be ∼ 0.3 μm s −1 , consistent with the bulk data. This result clearly indicates that     one can control the orientation of the one-dimensional motion of bound beads by     manipulating the alignment of nanofibre 1 . The results presented here show that a fluidic supramolecular nanofibre can function as an artificial molecular rail for converting the three-dimensional random motion of attached substrates such as lipids, proteins and nanobeads into one-dimensional mode. In addition, we can intentionally guide the one-dimensional motion along the aligned fibre in a microchannel because of the elastic toughness and flexibility of the nanofibre. We determined that the averaged speed was ∼ 0.3 μm s −1 , which is controlled by the lipid mobility in    the fluidic fibre, independent of bead size. Interestingly, although the transport mechanism    is completely different, this is almost identical to the speed of microtubule-binding     proteins [20] and DNA-binding proteins [22] without     ATP energy diffusing along    microtubules and DNA (0.1–0.4 μm 2 s −1 ), respectively, and is    slightly lower than that of kinesin moving on microtubules (about 1 μm s −1 )    powered by the energy of ATP     hydrolysis [54] . Therefore, it is clear that the present artificial system,    which uses lipid fluidity in the nanofibre without chemical energy, can produce a cargo    speed comparable with that of biological diffusional motility systems. The directionality of    movement cannot be regulated in the present system unlike the one-directional motion of    kinesin along microtubules. However, we believe that this is an important first step in the    construction of artificial mass transporting systems that can work at the micrometre    scale. Supramolecular fibre preparation and CLSM observations A suspension of glycolipid 1 or 2 (1.0 mg, 0.25 wt%) in water (396 μl) was heated to form a     homogeneous solution. To this solution was added a solution of fluorescent probe      (ANS) in methanol and the resulting mixture was     gently shaken. The solution (10 μl) was spotted on a glass-bottom dish (Matsunami,     non-coat, 0.15–0.18 mm glass bottom), incubated to complete gelation in a sealed box with     high humidity at room temperature for 1 h. The sample was then subjected to CLSM     observation using an inverted CLSM (Olympus      FV1000-ASW, Olympus) equipped with a 543 and 633 nm     Helium Neon, a 488 nm multi-Ar laser (Coherent). A ×100, NA=1.40 oil objective or a ×10, NA=0.40 air     objective was used to obtain images. TEM and SEM observations A suspension of glycolipid 1 (1.0 mg, 0.25 wt%) in distilled water (400 μl) was     heated to form a homogeneous solution and the solution was cooled to room temperature. The     solution (5 μl) was spotted on a copper TEM grid covered by an elastic carbon-support film     (20–25 nm) with a filter paper underneath, and excess solution was blotted immediately     with filter paper. The TEM grid was dried under a reduced pressure for at least 6 h before     TEM observation. No coating or staining was applied for TEM observation. TEM images were     acquired using a JEOL     JEM-1025 (accelerating voltage, 100 kV) equipped     with a CCD camera. SEM samples were prepared by casting the solution on a silicon wafer     and dried under reduced pressure for at least 6 h. Platinum was then sputtered on the     dried sample for 90 s using a JEOL     JFC-1600. SEM images were acquired using a JEOL     JSM-5600B (accelerating voltage, 15–20 kV) equipped     with a CCD camera. PDMS device fabrication A mould of PDMS was formed by curing the prepolymer (Sylgard 184; Dow Corning) on a 2-inch silicon wafer     master having a positive relief (50 μm) of the capillary channels formed in a photoresist     (SU-8) on its surface. The peeled-off PDMS mould was placed on a cover glass (Matsunami,     non-coat, 0.15–0.18 mm glass bottom) and used without permanent bonding. FRAP study of supramolecular fibres A glycolipid 1 (1.0 mg) was suspended in 50 mM HEPES (4-(2-hydroxyethyl)-1-piperazineethanesulfonic      acid) buffer (pH 7.2, 396 μl), and the mixture was then heated to form     a homogeneous solution. To this solution, a solution of fluorescent probe (4.0 μl) in     methanol was added and the resulting mixture was gently shaken. The mixture (10 μl) was     spotted on the cover glass of a dish for CLSM observation and incubated in a sealed box     with high humidity at room temperature for 1 h. After a small area of the fibres was     viewed on CLSM, the fluorescein moiety of FITC-lipid 3 in this region was photobleached by an intense Ar     laser irradiation (488 nm). The fluorescence image of the same area was continuously     monitored in real time using a low level of the monitoring light to suppress further     photobleaching. The obtained time-lapse images were analysed with software embedded in a     microscope and using ImageJ 1.38 on a Macintosh PC. After importing the data into KaleidaGraph 4.0 (Synergy),     each intensity profile was fitted to a Gaussian function and the obtained time decay was     curve fitted with a one-dimensional diffusion equation ( Fig. 4a,b , Supplementary Fig. S4 ). Electrically controlled transport study of supramolecular fibres In this experiment, the solution of supramolecular nanofibres 1 / 3 + 4 prepared as described above was mixed with agarose (4 wt%) to restrict the electrophoretic     migration of the nanofibre. The homogeneous mixture containing supramolecular nanofibres 1 / 3 + 4 and agarose was introduced into a microchannel     (width×height=150×50 μm) of PDMS and the sample was then incubated at room temperature for     1 h. Both ends of the microchannel were sealed by agarose gel to prevent drying and were     placed in contact with the electrode. The electric field (15 V cm −1 ) was     applied and the movements of the fluorescent probes were traced on CLSM. Tracing nanobeads attached to supramolecular fibres A suspension of glycolipid 1 (1.0 mg, 0.10 wt%) in distilled water (1.0 ml) was     heated to form a homogeneous solution. To this warm solution (50 μl) was added a DMSO     solution (2.5 μl) of biotin-lipid 5 (0.50 mM) and the resulting mixture was gently     shaken and incubated at room temperature for 5 min. To this mixture was added a suspension     of SA beads (1.0 wt%, 2.0 μl), and the sample was then subjected to CLSM observation. The     trajectories of the beads were tracked with Move-tr/2D      7.0 software (Library) on a Windows PC. How to cite this article: Tamaru, S.-i. et al . Fluidic supramolecular nano-    and micro-fibers as molecular rails for regulated movement of nanosubstances. Nat. Commun. 1:20 doi: 10.1038/ncomms1018 (2010).